A functional deficiency of TERA/VCP/p97 contributes to impaired DNA repair in multiple polyglutamine diseases It is hypothesized that a common underlying mechanism links multiple neurodegenerative disorders. Here we show that transitional endoplasmic reticulum ATPase (TERA)/valosin-containing protein (VCP)/p97 directly binds to multiple polyglutamine disease proteins (huntingtin, ataxin-1, ataxin-7 and androgen receptor) via polyglutamine sequence. Although normal and mutant polyglutamine proteins interact with TERA/VCP/p97, only mutant proteins affect dynamism of TERA/VCP/p97. Among multiple functions of TERA/VCP/p97, we reveal that functional defect of TERA/VCP/p97 in DNA double-stranded break repair is critical for the pathology of neurons in which TERA/VCP/p97 is located dominantly in the nucleus in vivo . Mutant polyglutamine proteins impair accumulation of TERA/VCP/p97 and interaction of related double-stranded break repair proteins, finally causing the increase of unrepaired double-stranded break. Consistently, the recovery of lifespan in polyglutamine disease fly models by TERA/VCP/p97 corresponds well to the improvement of double-stranded break in neurons. Taken together, our results provide a novel common pathomechanism in multiple polyglutamine diseases that is mediated by DNA repair function of TERA/VCP/p97. Transitional endoplasmic reticulum (ER) ATPase (TERA), also known as valosin-containing protein (VCP) or p97, is implicated in various neurodegenerative disorders. Mutations in the human TERA/VCP/p97 gene cause frontotemporal dementia associated with inclusion body myopathy and early-onset Paget disease [1] or familial amyotrophic lateral sclerosis [2] , and TERA/VCP/p97 is now considered a major causative gene for frontotemporal lobar degeneration (FTLD). The TERA/VCP/p97 protein also interacts with a normal length polyglutamine (polyQ) tract sequence derived from a transcription factor, Brn-2 (ref. 3 ), and the mutant form of a polyglutamine disease protein, ataxin-3 (ref. 4 ), which causes spinocerebellar ataxia type 3. TERA/VCP/p97 is a member of the ATPase associated with various activities AAA+ protein family involved in diverse cellular functions. The name TERA is derived from its function in the membrane transfer from the ER to the Golgi apparatus. TERA/VCP/p97 contains ATPase catalytic domains and regulatory N-terminal and C-terminal domains; it forms a hexameric structure and couples ATP hydrolysis to cellular activities [5] . For instance, the budding process of transition vesicles from smooth and rough ER is ATP-dependent and requires TERA/VCP/p97 (ref. 6 ). TERA/VCP/p97 is essential for cistern reformation from mitotic Golgi fragments [7] . TERA/VCP/p97 also interacts with clathrin [8] , which coats the endosome membrane. TERA/VCP/p97 has a critical role in ER-associated protein degradation (ERAD) though interactions with Derlin-1, VCP-interacting membrane protein [9] and UFD1/NPL4 complex [10] . TERA/VCP/p97 supplies energy to this protein complex to extract misfolded proteins from the ER lumen and transport them to the proteasome for degradation. TERA/VCP/p97 may directly interact with gp78, a sensor of misfolded proteins, on the ER membrane [11] , and may also interact with small interfering RNA to affect cell division [12] . Furthermore, a recent report revealed a role of TERA/VCP/p97 in DNA double-stranded break (DSB) repair, as TERA/VCP/p97 interacts with and promotes release of lethal (3) malignant brain tumor-like protein 1 (L3MBTL1) from DSBs and recruitment of p53-binding protein-1 (53BP1) [13] , [14] . Hence, TERA/VCP/p97 regulates ERAD, membrane transport and DSB repair. Despite these findings, it remains unclear how TERA/VCP/p97 is altered in FTLD or motor neuron disease associated with TERA/VCP/p97 gene mutations. RNAi-mediated depletion of TERA/VCP/p97 induces accumulation of ubiquitinated proteins, vacuolization of ER, impairment of protein trafficking through the secretory pathway, and induces apoptosis in cell lines [15] , [16] , [17] . However, overexpression of mutant TERA/VCP/p97 causes degeneration phenotypes in vitro [18] and in vivo [19] , [20] , [21] . ATPase activity was increased in some experiments using the GST-TERA/VCP/p97 fusion protein [22] , [23] . In spinocerebellar ataxia type 3, mutant ataxin-3 changes TERA/VCP/p97 modification, promotes nuclear translocation of TERA/VCP/p97, and suppresses transcription [24] , suggesting a pathological role of TERA/VCP/p97 in the nucleus. Like FTLD, these results have not yet been verified, and it is unclear how ATPase or ERAD activities and the other functions of TERA/VCP/p97 are affected in neurodegeneration. Our previous observation that TERA/VCP/p97 physically interacts with the polyQ sequence [3] prompted us to revisit the question whether TERA/VCP/p97 has a common pathological role in multiple polyQ diseases. As expected, we show that multiple polyQ disease proteins for bulbospinal muscular atrophy/Kennedy’s disease, spinocerebellar ataxia type 1 (SCA1), spinocerebellar ataxia type 7, and Huntington’s disease (HD) physically interact with TERA/VCP/p97. Though TERA/VCP/p97 binds to normal as well as mutant polyQ proteins, mutant polyQ proteins specifically affect dynamism of TERA/VCP/p97 and impair its function. Mislocalization of TERA/VCP/p97 to aggregates is confirmed in diseased human brains. More surprisingly, TERA/VCP/p97 is localized to the nucleus in human and mouse adult neuron in vivo . Live imaging reveals that mutant polyQ proteins specifically impair recruitment of TERA/VCP/p97 to DNA damage foci and inhibit DSB repair. Suppression of ERAD is relatively weak in primary neurons from mutant ATXN1-knock in (KI) mice. TERA/VCP/p97 genetically rescues phenotypes in Drosophila HD and SCA1 models in consistence with the recovery of DSB. Taken together, we propose a novel hypothesis that impairment of TERA/VCP/p97-mediated DSB repair is a common pathology in multiple polyQ diseases. Mutant and normal polyQ proteins interact with TERA/VCP/p97 We performed an immunoprecipitation (IP) assay to test interaction between TERA/VCP/p97 and polyQ disease proteins. TERA/VCP/p97 was co-expressed in HeLa cells with full-length ataxin-1 (ATXN1), huntingtin exon 1 (Htt-exon1), full-length ataxin-7 (ATXN7) or androgen receptor (AR) by expression vectors. TERA/VCP/p97 was tagged with FLAG, while the polyQ proteins were tagged with Myc-peptide. Both anti-Myc and anti-FLAG antibodies co-precipitated the counterpart ( Fig. 1 ). The affinity was different for the various polyQ proteins; ATXN1 and Htt-exon1 were bound tightly to TERA/VCP/p97 ( Fig. 1a ), whereas interaction between ATXN7 and TERA/VCP/p97 seemed weak ( Fig. 1a ). However, beyond such differences, all polyQ proteins bound to TERA/VCP/p97. In the same IP condition, we could never found binding of c-Jun, c-Fos or RIP1 to polyQ proteins in multiple trials ( Supplementary Fig. S1 ). Surprisingly, both normal as well as mutant polyQ proteins interacted with TERA/VCP/p97 in all instances, although the affinity of mutant polyQ protein was basically higher ( Fig. 1a ). The affinity to the soluble form of mutant polyQ protein was basically higher, except in the case of Htt-exon1-103Q protein where insoluble (bar in Fig. 1a ) rather than soluble proteins (arrow in Fig. 1a ) were sticky to TERA/VCP/p97. Multiple bands of polyQ proteins corresponded to different states of aggregation from monomer to polymer and/or different protein structures. 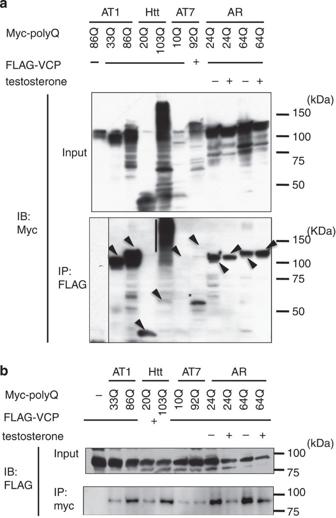Figure 1: Multiple polyQ proteins interact with TERA/VCP/p97. (a) VCP coprecipitates with normal as well as mutant forms of ataxin-1 (ATXN1), huntingtin (Htt), full-length ataxin-7 (ATXN7) or androgen receptor (AR). HeLa cells were co-transfected with Myc-polyQ and FLAG-VCP protein expression vectors, and the cell lysates were immunoprecipitated with anti-FLAG antibody. Lane 1 is a negative control in which HeLa cells are transfected with Myc-ATXN1-86Q expression vector only. Coprecipitation of ATXN7 is relatively unstable. AR binds strongly to VCP in the absence of testosterone (T−) but only weakly in the presence of testosterone (T+) because of the dissociation of their intracellular distribution. Arrows indicate co-precipitated full-length proteins, and bar indicates co-precipitated Htt aggregates. (b) Normal and mutant polyQ proteins coprecipitate with VCP. ATXN7 did not obviously coprecipitate in some cases. Mutant Htt seems to bind more strongly to VCP than to normal Htt in these blots; however, the difference is not definite in other blots. Figure 1: Multiple polyQ proteins interact with TERA/VCP/p97. ( a ) VCP coprecipitates with normal as well as mutant forms of ataxin-1 (ATXN1), huntingtin (Htt), full-length ataxin-7 (ATXN7) or androgen receptor (AR). HeLa cells were co-transfected with Myc-polyQ and FLAG-VCP protein expression vectors, and the cell lysates were immunoprecipitated with anti-FLAG antibody. Lane 1 is a negative control in which HeLa cells are transfected with Myc-ATXN1-86Q expression vector only. Coprecipitation of ATXN7 is relatively unstable. AR binds strongly to VCP in the absence of testosterone (T−) but only weakly in the presence of testosterone (T+) because of the dissociation of their intracellular distribution. Arrows indicate co-precipitated full-length proteins, and bar indicates co-precipitated Htt aggregates. ( b ) Normal and mutant polyQ proteins coprecipitate with VCP. ATXN7 did not obviously coprecipitate in some cases. Mutant Htt seems to bind more strongly to VCP than to normal Htt in these blots; however, the difference is not definite in other blots. Full size image The interaction with AR was remarkably reduced in testosterone (50 nM, 24 h)-treated cells (T+), suggesting that nuclear translocation of ligand-bound AR decreases the chance of association with TERA/VCP/p97 localized to the cytoplasm in HeLa cells. Consistent with our previous observation [3] , deletion of the polyQ tract by using Htt, ATXN1, ATXN7 and AR remarkably decreased their affinities to TERA/VCP/p97 ( Supplementary Fig. S2 ), indicating that interaction between polyQ and TERA/VCP/p97 is based on the polyQ tract sequence. Mutant polyQ proteins mislocalize TERA/VCP/p97 We next addressed how interaction influences subcellular localization of TERA/VCP/p97. As neurons are not suitable for detailed analysis of cytoplasmic localization, we used HeLa cells with larger cytoplasm. Mutant ATXN1, AR(T+) and Htt-exon1 proteins formed either nuclear or cytoplasmic inclusion bodies at high frequency ( Fig. 2a ). As expected from the biochemical interaction ( Fig. 1 ), TERA/VCP/p97 was co-localized with most of the polyQ proteins ( Fig. 2a ). In such aggregate-positive cells, TERA/VCP/p97 was sequestered to the inclusion bodies (ATXN1-86Q, Htt-103Q and AR-64Q T+) and its subcellular distribution was shifted ( Fig. 2b ). Filter-binding assay supported the sequestration of TERA/VCP/p97 by mutant polyQ proteins ( Fig. 2c ), and unbound TERA/VCP/p97 (=membrane filtered) was reduced by mutant polyQ proteins in a dose-dependent manner ( Supplementary Fig. S3 ). 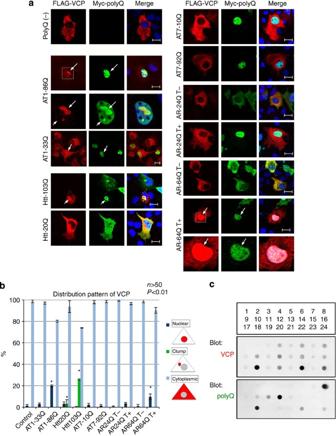Figure 2: Mutant polyQ proteins sequester TERA/VCP/p97 into the inclusion body. (a) HeLa cells co-transfected with Myc-polyQ and FLAG-VCP protein expression vectors are stained with anti-FLAG and anti-Myc antibodies. The top panels show normal cytoplasmic distribution of the FLAG-VCP protein. The ATXN1-86Q and Htt-103Q proteins sequester VCP to nuclear and cytoplasmic inclusion bodies, respectively. In contrast, the ATXN1-33Q and Htt-20Q proteins do not affect the cytoplasmic distribution of VCP regardless of their interaction. Normal and mutant ATXN7 expression did not affect intracellular localization of VCP. In the presence of testosterone, mutant but not normal AR sequesters VCP into the nucleus. Scale bar, 20 μm. (b) Quantitative analysis of the change of intracellular distribution of VCP by polyQ proteins. The distribution patterns are described in right panels. Means and s.e.m. are indicated. Asterisks indicate statistical difference from the control (P<0.01, Student’st-test). (c) Filter-binding assay shows co-aggregation of polyQ disease proteins and VCP. 1, 2: buffer, 3 empty plasmid, 4: empty plasmid+VCP, 5: ATXN1-33Q, 6: ATXN1-33Q+VCP, 7: ATXN1-86Q, 8: ATXN1-86Q+VCP, 9: Htt-20Q, 10: Htt-20Q+VCP, 11: Htt-103Q, 12: Htt-103Q+VCP, 13: ATXN7-10Q, 14: ATXN7-10Q+VCP, 15: ATXN7-92Q, 16: ATXN7-92Q+VCP, 17: AR-24Q testosterone (−), 18: AR-24Q+VCP testosterone (−), 19: AR-24Q testosterone (+), 20: AR-24Q+VCP testosterone (+), 21: AR-64Q testosterone (−), 22: AR-64Q+VCP testosterone (−), 23: AR-64Q testosterone (+), 24: AR-64Q+VCP testosterone (+). Figure 2: Mutant polyQ proteins sequester TERA/VCP/p97 into the inclusion body. ( a ) HeLa cells co-transfected with Myc-polyQ and FLAG-VCP protein expression vectors are stained with anti-FLAG and anti-Myc antibodies. The top panels show normal cytoplasmic distribution of the FLAG-VCP protein. The ATXN1-86Q and Htt-103Q proteins sequester VCP to nuclear and cytoplasmic inclusion bodies, respectively. In contrast, the ATXN1-33Q and Htt-20Q proteins do not affect the cytoplasmic distribution of VCP regardless of their interaction. Normal and mutant ATXN7 expression did not affect intracellular localization of VCP. In the presence of testosterone, mutant but not normal AR sequesters VCP into the nucleus. Scale bar, 20 μm. ( b ) Quantitative analysis of the change of intracellular distribution of VCP by polyQ proteins. The distribution patterns are described in right panels. Means and s.e.m. are indicated. Asterisks indicate statistical difference from the control ( P <0.01, Student’s t -test). ( c ) Filter-binding assay shows co-aggregation of polyQ disease proteins and VCP. 1, 2: buffer, 3 empty plasmid, 4: empty plasmid+VCP, 5: ATXN1-33Q, 6: ATXN1-33Q+VCP, 7: ATXN1-86Q, 8: ATXN1-86Q+VCP, 9: Htt-20Q, 10: Htt-20Q+VCP, 11: Htt-103Q, 12: Htt-103Q+VCP, 13: ATXN7-10Q, 14: ATXN7-10Q+VCP, 15: ATXN7-92Q, 16: ATXN7-92Q+VCP, 17: AR-24Q testosterone (−), 18: AR-24Q+VCP testosterone (−), 19: AR-24Q testosterone (+), 20: AR-24Q+VCP testosterone (+), 21: AR-64Q testosterone (−), 22: AR-64Q+VCP testosterone (−), 23: AR-64Q testosterone (+), 24: AR-64Q+VCP testosterone (+). Full size image Distribution pattern of TERA/VCP/p97 was remarkably changed in cells co-expressing mutant ATXN1, AR or Htt-exon1 proteins ( Fig. 2a ), while mutant ATXN7 did not remarkably shift TERA/VCP/p97 to the nucleus ( Fig. 2a ) agreeing with the weak binding between ATXN7 and TERA/VCP/p97 ( Fig. 1a ). It is of note that TERA/VCP/p97 in the nucleoplasm was substantially reduced in mutant ATXN1- or mutant Htt-expressing cells ( Fig. 2a ). In the case of mutant ATXN1-expressing cells, TERA/VCP/p97 was sequestered to nuclear inclusions and deprived from the nucleoplasm ( Fig. 2a ), while the deprivation was unclear in mutant AR(T+) cells with homogeneous nuclear aggregates ( Fig. 2a ). Meanwhile, intracellular distribution of TERA/VCP/p97 was not changed by normal polyQ proteins ( Fig. 2a ); instead, it was consistent with a low affinity to TERA/VCP/p97 in the case of ATXN7 or with the cytoplasmic non-aggregating localization of the normal AR(T−) and Htt-exon1. However, in the case of normal ATXN1 and AR(T+) located in the nucleus, sequestration of TERA/VCP/p97 was not observed, despite the biochemical interaction. This might be due to a difference in biochemical composition between nuclear foci and nuclear inclusion bodies. Even in the case of nuclear inclusion bodies, reports have shown that polyQ proteins dynamically shuttle in and out of the inclusion bodies and that the shuttling speed is dependent on polyQ length [25] , [26] , [27] . Presumably, sequestration can occur only when TERA/VCP/p97 is bound tightly to the inside structure of such aggregates. Mutant polyQs impair DSB repair function of TERA/VCP/p97 TERA/VCP/p97 have multiple functions like protein transport from ER to the plasma membrane, ERAD and recently identified DSB repair [13] , [14] . Surprisingly, immunohistochemistry with multiple anti-VCP antibodies revealed that TERA/VCP/p97 is localized dominantly in the nucleus of adult neurons ( Supplementary Fig. S4 ) contrastively to the cytoplasmic localization in hepatocytes or renal tubules cells ( Supplementary Fig. S5 ). Furthermore, the nuclear dominant distribution of TERA/VCP/p97 was confirmed in normal human neurons including vulnerable subtypes in polyQ diseases ( Supplementary Fig. S6 ). The result clearly indicated that nuclear function of TERA/VCP/p97 is more important than the other cytoplasmic functions, in human and mouse adult neurons. Therefore, we firstly tested whether sequestration of TERA/VCP/p97 impairs DSB repair. Immunohistochemistry with human patient brains of HD and SCA1 revealed that TERA/VCP/p97 was depleted from the nucleoplasm in affected neurons by sequestration to cytoplasmic (perinuclear) or nuclear inclusion bodies ( Fig. 3a ). In human HD brains, TERA/VCP/p97 was co-localized with mutant Htt in the marginal zone of the nucleus or in the perinuclear cytoplasmic region of striatal neurons ( Fig. 3a , upper panels); however, TERA/VCP/p97 was sometimes concentrated in the cleft, where the cytoplasm is inserted into the nucleus in cortical neurons ( Fig. 3a , middle panels). In human SCA1 brains, TERA/VCP/p97 was co-localized in nuclear inclusions of Purkinje cells or occasionally in shrunken nuclei of cerebellar granule cells ( Fig. 3a , lower panels). In all cases, signals of TERA/VCP/p97 were very low in the nucleoplasm. 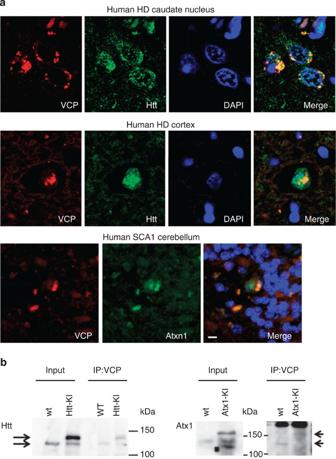Figure 3: Mutant polyQ proteins interact with TERA/VCP/p97 in the human brain. (a) Mutant polyQ proteins and VCP are co-localized in inclusion bodies of human patients with polyQ diseases. Subcellular distribution of VCP was remarkably changed in neurons possessing aggregates of polyQ disease proteins. Scale bar, 10 μm. In control human brains, subcellular accumulation or foci of TERA/VCP/p97 was not observed (Supplementary Fig. S6). (b) Coprecipitation of mutant polyQ and VCP proteins from mutant polyQ-KI mouse brain samples. Figure 3: Mutant polyQ proteins interact with TERA/VCP/p97 in the human brain. ( a ) Mutant polyQ proteins and VCP are co-localized in inclusion bodies of human patients with polyQ diseases. Subcellular distribution of VCP was remarkably changed in neurons possessing aggregates of polyQ disease proteins. Scale bar, 10 μm. In control human brains, subcellular accumulation or foci of TERA/VCP/p97 was not observed ( Supplementary Fig. S6 ). ( b ) Coprecipitation of mutant polyQ and VCP proteins from mutant polyQ-KI mouse brain samples. Full size image Interaction between polyQ proteins and TERA/VCP/p97 in vivo and sequestration of TERA/VCP/p97 into aggregates were also confirmed by IP ( Fig. 3b ) and immunohistchemsitry ( Supplementary Fig. S7 ) with brains from model mice. We used KI mouse brain tissues from full-length mutant Htt-111Q [28] or mutant ATXN1-154Q [29] , together with mutant Htt- [30] , ATXN7- [31] or AR-transgenic (Tg) mice [32] . Again we confirmed the co-localization of mutant polyQ proteins with TERA/VCP/p97 in Htt-Tg (R6/2), Htt-KI, ATXN1-KI and AR-Tg mice ( Supplementary Figs S7a–c, S8 ). In ATXN7-Tg mice in which ATXN7 is expressed just above the endogenous level [31] , sequestration of VCP to the inclusion body was not obvious ( Supplementary Fig. S7d ). In Htt-Tg (R6/2), Htt-KI, ATXN1-KI and AR-Tg mice, TERA/VCP/p97 was decreased in the nucleoplasm when compared with their controls ( Supplementary Fig. S8 ). An IP assay also confirmed endogenous interaction between mutant Htt and TERA/VCP/p97 in HD model mice ( Fig. 3b ). Moreover, we tested whether mutant polyQ proteins impair the dynamics of TERA/VCP/p97 to DSB lesions induced by high-energy UVA ( Supplementary Fig. S9 ). In U2OS cells expressing Atxn1-86Q-DsRed, accumulation of VCP-EGFP to the DSB lesion was slowed down in comparison with Atxn1-33Q-DsRed-expressing cells or mock-treated cells ( Fig. 4a ). In the case of mutant Htt expression, the delay was also remarkable in the cells possessing DsRed signals of Htt-103Q in the nucleus even without nuclear inclusion body ( Fig. 4a ), suggesting that pre-aggregates of mutant Htt impaired dynamics of TERA/VCP/p97 to nuclear DSB lesions. However, the delay of VCP-EGFP accumulation became more profound when inclusion bodies were formed in Atxn1-86Q-DsRed or Htt-103Q-DsRed expressing cells ( Fig. 4a ), indicating that aggregation also contributes to the delay. 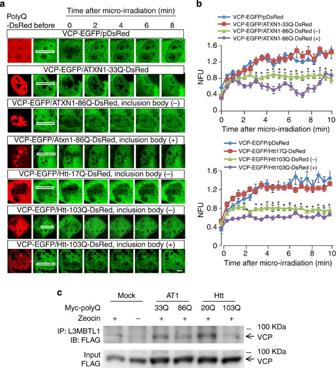Figure 4: Mutant polyQ proteins delay accumulation of TERA/VCP/p97 to DSB foci. (a) Sequential images showing accumulation of VCP-EGFP to the linear DSB. In cells expressing mutant polyQ proteins (Atxn1-86Q-DsRed and Htt-103Q-DsRed), the accumulation of VCP-EGFP was delayed in comparison with non-transfected or normal polyQ protein (Atxn1-33Q-DsRed and Htt-17Q-DsRed) expressing cells. Among the cells expressing mutant polyQ proteins, the delay in the accumulation of VCP-EGFP was more remarkable in inclusion body-positive cells than in inclusion body-negative cells. Scale bar, 5 μm. (b) Quantitative analysis of the recovery of VCP-EGFP signals at the linear photobleach areas that correspond to accumulation of VCP-EGFP to the DSB lesion (N=6). The signals were obtained from more than four sites on the linear damage area, and the mean value was used for the quantitative analyses at each time point. Means and s.e.m. are indicated. Asterisks indicate statistical difference from the value of normal polyQ protein-expressing cells at the same time point (P<0.01, Student’st-test). H2Ax staining confirmed that DSB was actually induced in this condition (Supplementary Fig. 8). NFU: normalized fluorescence unit. (c) Mutant polyQ proteins inhibit interaction between TERA/VCP/p97 and L3MBTL1. Zeocin (400 μg ml−1) was added to the culture medium of HeLa cells to induce DSBs where TERA/VCP/p97 interacts with L3MBTL1. Mutant Htt and ATXN1 both decrease the interaction between TERA/VCP/p97 and L3MBTL1. Figure 4: Mutant polyQ proteins delay accumulation of TERA/VCP/p97 to DSB foci. ( a ) Sequential images showing accumulation of VCP-EGFP to the linear DSB. In cells expressing mutant polyQ proteins (Atxn1-86Q-DsRed and Htt-103Q-DsRed), the accumulation of VCP-EGFP was delayed in comparison with non-transfected or normal polyQ protein (Atxn1-33Q-DsRed and Htt-17Q-DsRed) expressing cells. Among the cells expressing mutant polyQ proteins, the delay in the accumulation of VCP-EGFP was more remarkable in inclusion body-positive cells than in inclusion body-negative cells. Scale bar, 5 μm. ( b ) Quantitative analysis of the recovery of VCP-EGFP signals at the linear photobleach areas that correspond to accumulation of VCP-EGFP to the DSB lesion ( N =6). The signals were obtained from more than four sites on the linear damage area, and the mean value was used for the quantitative analyses at each time point. Means and s.e.m. are indicated. Asterisks indicate statistical difference from the value of normal polyQ protein-expressing cells at the same time point ( P <0.01, Student’s t -test). H2Ax staining confirmed that DSB was actually induced in this condition ( Supplementary Fig. 8 ). NFU: normalized fluorescence unit. ( c ) Mutant polyQ proteins inhibit interaction between TERA/VCP/p97 and L3MBTL1. Zeocin (400 μg ml −1 ) was added to the culture medium of HeLa cells to induce DSBs where TERA/VCP/p97 interacts with L3MBTL1. Mutant Htt and ATXN1 both decrease the interaction between TERA/VCP/p97 and L3MBTL1. Full size image We also tested the TERA/VCP/p97 dynamics after microirradiation in primary mouse cortical neurons. As primary neurons have too small nuclei for high-energy damage and they were highly vulnerable to suffer some levels of DNA damages during primary culture, we used lentiviral vectors for expression of polyQ proteins, reduced the energy of microirradiation and performed signal acquisition by immunocytochemistry at 1 h after microirradiation. Accumulation of TERA/VCP/p97 to damaged area was also delayed in primary neurons expressing Atxn1-86Q-DsRed or Htt-103Q-DsRed in comparison with primary neurons expressing DsRed or normal polyQ proteins ( Fig. 5a ). 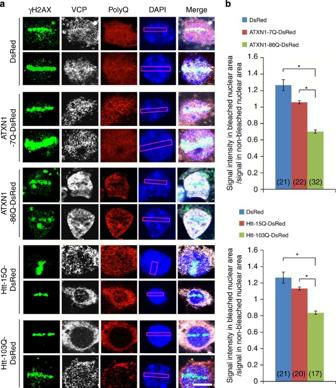Figure 5: Delayed dynamics of TERA/VCP/p97 recruitment to DSBs by mutant polyQ proteins in primary cortical neurons. (a) The fluorescent signal of TERA/VCP/p97 at DSBs was decreased in Atxn1-86Q-DsRed or Htt-103Q-DsRed expressing mouse primary cortical neurons more than the control neurons expressing DsRed, Atxn1-7Q-DsRed or Htt-15Q-DsRed at 1 h after laser microirradiation. Signals of TERA/VCP/p97 were obtained from γH2AX-positive bleached area. Scale bar, 5 μm. (b) The signal intensity in bleached nuclear area/signal in non-bleached nuclear area was decreased in mutant polyQ expressing neurons more than the control neurons. Means and s.e.m. are indicated. Asterisks indicate statistical difference of the value between control neurons and polyQ protein-expressing neurons (P<0.01, Student’st-test). Figure 5: Delayed dynamics of TERA/VCP/p97 recruitment to DSBs by mutant polyQ proteins in primary cortical neurons. ( a ) The fluorescent signal of TERA/VCP/p97 at DSBs was decreased in Atxn1-86Q-DsRed or Htt-103Q-DsRed expressing mouse primary cortical neurons more than the control neurons expressing DsRed, Atxn1-7Q-DsRed or Htt-15Q-DsRed at 1 h after laser microirradiation. Signals of TERA/VCP/p97 were obtained from γH2AX-positive bleached area. Scale bar, 5 μm. ( b ) The signal intensity in bleached nuclear area/signal in non-bleached nuclear area was decreased in mutant polyQ expressing neurons more than the control neurons. Means and s.e.m. are indicated. Asterisks indicate statistical difference of the value between control neurons and polyQ protein-expressing neurons ( P <0.01, Student’s t -test). Full size image TERA/VCP/p97 interacts with L3MBTL1, facilitates replacement of L3MBTL1 with 53BP1, changes the chromatin for DSB repair [13] . Therefore, we tested whether mutant polyQ proteins disturbed this process. Consistently with the impaired dynamics of TERA/VCP/p97 in the nucleus, both ATXN1-86Q and Htt-103Q proteins inhibited interaction between transfected VCP-FLAG and endogenous L3MBTL1 ( Fig. 4c ). Moreover, extraction of L3MBTL1 from the linear DSB lesion and replacement with 53BP1 were actually delayed at an early time point after microirradiation ( Supplementary Fig. S10a,b ). Consequently, the signal intensities of γH2Ax remained at higher levels in U2OS cells expressing Atxn1-86Q-DsRed or Htt-103Q-DsRed ( Supplementary Fig. S10c ). The nuclear situation in U2OS cells could be analogous to polyQ disease mouse models in which TERA/VCP/p97 was deprived from nucleoplasm to inclusion bodies ( Supplementary Figs 7,8 ). It could explain the remarkable increase of DSB in polyQ disease mouse models ( Supplementary Fig. S11 ). High γH2Ax signals were observed predominantly in vulnerable neurons of each mouse model ( Fig. 6 ) and correlated with sequestration or disappearance of TERA/VCP/p97 ( Supplementary Fig. S12 ). 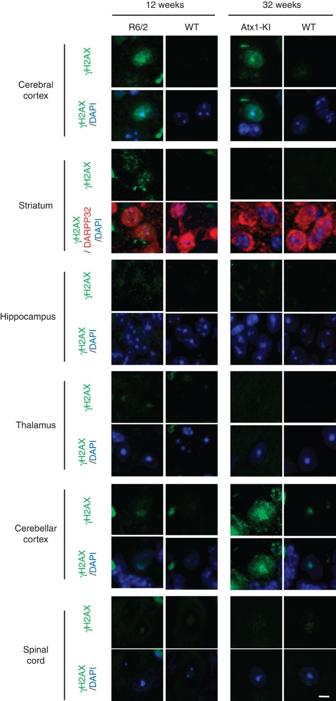Figure 6: DSBs are prominent in vulnerable types of neurons. Various brain regions of R6/2 (12 weeks) and Atxn1-KI mice (32 weeks) were stained with γH2AX antibody. The controls (WT) were age-matched littermates. DARPP32 is a marker of medium spiny neurons. Scale bar, 5 μm. Figure 6: DSBs are prominent in vulnerable types of neurons. Various brain regions of R6/2 (12 weeks) and Atxn1-KI mice (32 weeks) were stained with γH2AX antibody. The controls (WT) were age-matched littermates. DARPP32 is a marker of medium spiny neurons. Scale bar, 5 μm. Full size image Mutant polyQs affect ER-related functions of TERA/VCP/p97 Although the nuclear function of TERA/VCP/p97 was implicated in the polyQ disease pathology, involvement of the other functions of TERA/VCP/p97 cannot be excluded. Therefore, we tested whether mislocalization or sequestration influenced the other cytoplasmic functions of TERA/VCP/p97 like protein transport and ERAD. In the first case, dominant-negative TERA/VCP/p97 (VCP-DN) was known to impair transport of ErbB2 protein from ER to the plasma membrane [33] . They reported that ErbB2 could not pass the quality control system and accumulated around the nucleus [33] . As expected, when mutant polyQ proteins were expressed in HeLa cells, EGFP-ErbB2 was stacked in the perinuclear region ( Supplementary Fig. S13a ). AR-64Q induced similar accumulation irrespective of testosterone ( Supplementary Fig. S13a ). TERA/VCP/p97 co-expression recovered the ErbB2 perinuclear accumulation ( Supplementary Fig. S13b,c ). Mutant polyQ proteins also increased cytoplasmic vacuoles co-stained with an ER marker but distinct from autophagosomes ( Supplementary Fig. S14a,b ). Moreover, we analysed primary mouse cortical neurons transfected by polyQ-DsRed and VCP-EGFP expression vectors. Co-localization of mutant polyQ and TERA/VCP/p97 proteins was confirmed ( Supplementary Fig. S15 ) like human or mouse disease brains ( Supplementary Figs S6, 7 ). In DsRed expressing neurons, VCP-EGFP was homogenously localized in the nucleus, while expression of Atxn1-86Q-DsRed changed the distribution heterogeneous in the nucleus and partially shifted to the cytoplasm ( Supplementary Fig. S15 ). Htt-103Q-DsRed clearly sequestered VCP-EGFP to inclusion bodies ( Supplementary Fig. S15 ). We also found that EGFP-ErbB2 was stacked around the nucleus in a part of primary neurons expressing mutant polyQ proteins ( Supplementary Fig. S16 ). Next, we investigated the effect of polyQ proteins on ERAD—an important function of TERA/VCP/p97—by using HEK293 cells and an ERAD substrate, CD3Δ. Expression vectors for Htt and ATXN1 proteins were co-transfected. When protein synthesis was blocked with cycloheximide (CHX), the actual amount of CD3Δ degradation by ERAD could be visualized ( Supplementary Fig. S17 ). Mutant but not normal Htt protein inhibited CD3Δ degradation significantly, whereas co-expression of TERA/VCP/p97 reverted CD3Δ accumulation by mutant Htt ( Supplementary Fig. S17a–c , left panels). Similar findings were observed in HeLa cells expressing the mutant ATXN1 protein ( Supplementary Fig. S17a–c , right panels). Further, to test the effect of mutant polyQ proteins on ERAD, we used primary cortical neurons prepared from Htt-111Q or ATXN1-154Q knock-in (KI) mice and tested CD3Δ degradation at 100 or 300 μg ml −1 CHX ( Supplementary Fig. S18 ). We confirmed that mutant Htt or ATXN1 expression disturbed ERAD at the endogenous expression level ( Supplementary Fig. S18a–c ); however, the effect was smaller than that observed in HeLa cells. Mutant polyQs weakly inhibit TERA/VCP/p97 ATPase activity We next determined whether mutant polyQ proteins affect the ATPase activity of TERA/VCP/p97. To do this, we used KI mice with the full-length human mutant Htt-111Q gene. We prepared from brain samples high molecular weight fractions corresponding to TERA/VCP/p97 immunoreactivity ( Supplementary Fig. S18d ). The fractions preserve the native hexamer of TERA/VCP/p97, which differs from the reconstructed TERA/VCP/p97 fusion protein produced in Escherichia coli cells, and we used it for an in vitro ATPase activity assay [22] , [34] . In this direct assay, ATPase activity of TERA/VCP/p97 per brain tissue weight was decreased in mutant Htt-KI mice ( Supplementary Fig. S18d ). We then examined the complex formation of TERA/VCP/p97 and Derlin-1 for protein quality control. According to the method described previously [9] , we tested the complex formation with brain samples from mutant Htt-KI mice. As expected, Derlin-1 co-precipitation with TERA/VCP/p97 in cortex was reduced ( Supplementary Fig. S18e ) indicating that interaction of TERA/VCP/p97 with mutant Htt inhibits the complex formation with Derlin-1. Taken together, the scheme obtained here was novel, and distinct from the previous one. This study revealed that mutant polyQ proteins suppressed ATPase activity of TERA/VCP/p97 in the brain tissue in vivo in contrast to the previous concept. Our results also suggested that non-cytoplasmic function of TERA/VCP/p97, that is, nuclear function of TERA/VCP/p97 is more critical for neurodegeneration. Mutant polyQ proteins suppressed dynamics of the nuclear TERA/VCP/p97 essential for DNA repair ( Fig. 4 , Supplementary Fig. S10 ) and increased DNA damage ( Fig. 6 , Supplementary Fig. S11 ). TERA/VCP/p97 rescues polyQ phenotypes in Drosophila Finally, we analysed whether TERA/VCP/p97 can rescue neurodegeneration phenotypes in vivo . For this analysis, we employed a new Drosophila model in which polyQ proteins are expressed specifically in motor neurons by the OK6 driver [35] . We used the GAL4–UAS system in which a transposon-containing upstream activation sequence (UAS) cis-element linked to a human polyQ gene is randomly integrated into the genome. We created UAS-Htt-103Q and UAS-ATXN1-85Q transgenic flies possessing a transgene integrated into chromosome 2. In the fly models, lifespan was shortened remarkably ( Fig. 7 ). We then mated the flies with TERA/VCP/p97 transgenic flies and observed the effect on the lifespan shortening. Consequently, TERA/VCP/p97 expression recovered the lifespan shortening of ATXN1-85Q and Htt-103Q transgenic flies ( Fig. 7 ). We confirmed equivalent expression levels of polyQ genes in the disease model and rescue flies by quantitative PCR ( Supplementary Fig. S19a ). Moreover, TERA/VCP/p97 restored the reduced thickness of the complex eye of the GMR-Gal4/UAS-ATXN1 fly ( Supplementary Fig. S19b,c ). 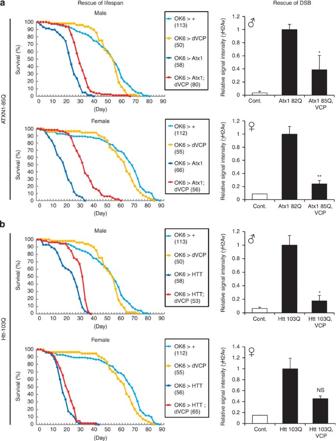Figure 7: TERA/VCP/p97 rescues lifespan shortening in mutant Htt and ATXN1 transgenic flies. Human Atxn1-85Q full-length protein (a) or Human Htt-103Q-exon1 peptide (b) expression in motor neurons by OK6-driver shortens the lifespan. Co-expression of VCP elongates the lifespan of both Atxn1 and Htt transgenic flies (log-rank test:P<0.01 in Atxn1 males and females and Htt males). The numbers of flies are shown after each fly genotype. Right graphs show the signals of γH2Av indicating double strand break (DSB) DNA damages. The signals were obtained from thoracic motor neurons (n=10–30/slide, 1 slide/fly, 5 flies/genotype), subtracted with background signals, and corrected by the number of neurons. The relative values were calculated as the ratio to the signals of mutant Atxn1 or Htt transgenic flies. Means and s.e.m. are indicated. *P<0.05, Student’st-test, **P<0.01, Student’st-test. Figure 7: TERA/VCP/p97 rescues lifespan shortening in mutant Htt and ATXN1 transgenic flies. Human Atxn1-85Q full-length protein ( a ) or Human Htt-103Q-exon1 peptide ( b ) expression in motor neurons by OK6-driver shortens the lifespan. Co-expression of VCP elongates the lifespan of both Atxn1 and Htt transgenic flies (log-rank test: P <0.01 in Atxn1 males and females and Htt males). The numbers of flies are shown after each fly genotype. Right graphs show the signals of γH2Av indicating double strand break (DSB) DNA damages. The signals were obtained from thoracic motor neurons ( n =10–30/slide, 1 slide/fly, 5 flies/genotype), subtracted with background signals, and corrected by the number of neurons. The relative values were calculated as the ratio to the signals of mutant Atxn1 or Htt transgenic flies. Means and s.e.m. are indicated. * P <0.05, Student’s t -test, ** P <0.01, Student’s t -test. Full size image Immunohistochemstry of motor neurons revealed that the extent of phenotype recovery was correlated well with the severity of DSB evaluated by staining with anti-γH2Av antibody in SCA1 fly models ( Fig. 7 right graph, Fig. 8 ). On the other hand, inclusion body formation of mutant Htt or diffuse nuclear accumulation of mutant ATXN1 was not largely affected by TERA/VCP/p97 ( Fig. 8 ). 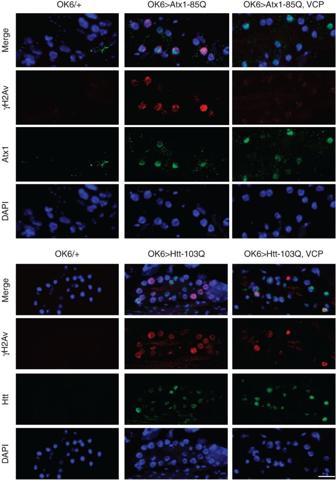Figure 8: TERA/VCP/p97 recovers DSBs in Drosophila motor neurons without affecting inclusion body formation. Drosophila thoracic motor neurons were co-stained with anti-γH2Av and anti-Atxn1(H21) or anti-Htt(N-18) antibodies. DSB detected by anti-γH2Av antibody was recovered by co-expression of VCP in SCA1 or Htt fly models, while inclusion body formation of mutant Htt or diffuse nuclear accumulation of mutant ATXN1 was not remarkably changed. Scale bar, 10 μm. Figure 8: TERA/VCP/p97 recovers DSBs in Drosophila motor neurons without affecting inclusion body formation. Drosophila thoracic motor neurons were co-stained with anti-γH2Av and anti-Atxn1(H21) or anti-Htt(N-18) antibodies. DSB detected by anti-γH2Av antibody was recovered by co-expression of VCP in SCA1 or Htt fly models, while inclusion body formation of mutant Htt or diffuse nuclear accumulation of mutant ATXN1 was not remarkably changed. Scale bar, 10 μm. Full size image Collectively, our results support that functional defect of TERA/VCP/p97 in DSB repair is a major factor contributing to neurodegeneration induced by mutant polyQ proteins in vivo . TERA/VCP/p97 is a multi-functional protein implicated in membrane traffic, cell cycle regulation, nuclear envelope reconstruction, ERAD, DNA damage repair and and autophagy [5] , [6] , [7] , [8] , [9] , [10] , [11] , [12] , [13] , [14] , [18] . Among such multiple functions, results in this study strongly suggest that functional defect of TERA/VCP/p97 in DSB repair underlies multiple polyQ diseases ( Supplementary Fig. S20 ). Mutant polyQ proteins impaired DSB repair by disturbing dynamics of TERA/VCP/p97 to DSB foci ( Fig. 4 ). Moreover, nuclear distribution of TERA/VCP/p97 in human adult neurons ( Supplementary Fig. S6 ), its sequestration into aggregates in human polyQ disease brains ( Fig. 3 ), and the tight link between in vivo phenotypes and DSBs ( Fig. 6 ) strongly supported that DSB repair mainly contributes to TERA/VCP/p97-mediated pathology in adult neurons. We reported previously that DNA repair molecules, HMGB1/2 and Ku70, were involved in HD and SCA1 [36] , [37] , which has recently been supported by the discovery of macroH2A—a human biomarker of HD [38] , [39] . This study added another DNA repair molecule, TERA/VCP/p97 to the pathology and further strengthened the DNA damage repair hypothesis of HD. In addition to TERA/VCP/p97’s function in DSB repair, some nuclear functions of TERA/VCP/p97 have been suspected. TERA/VCP/p97 interacts with the Aurora B kinase and regulates the reformation of the nucleus during the cell cycle [40] , and it might also act as a protein aggregation sensor that moves to the nucleus in response to protein aggregation [24] . As activation of cell cycle in neurodegeneration has been suggested by a number of results in non-dividing neurons [41] , [42] , [43] , our results do not exclude contribution of such nuclear functions of TERA/VCP/p97 to the polyQ disease common pathology. Presumably, such nuclear functions of TERA/VCP/p97 could be involved in the polyQ disease pathology, and further studies are necessary in the future. An increasing number of reports suggest that multiple polyQ diseases are partially based on common pathologies but also dependent on unique pathologies specific to each polyQ disease. Intriguingly, recent progress in interactome analysis and Drosophila genetics has contributed to this concept of common and unique pathologies [37] , [44] , [45] , [46] . Interactome analyses suggested that causative genes for polyQ diseases have mutually close relationships ( http://string-db.org/ )—a finding that was confirmed by genetic interaction in lower animal models [44] . Furthermore, comparison of transcriptome analysis data of multiple SCAs showed common signalling pathways [47] . This study supported the hypothesis through adding a new key player to the defect of DNA damage repair that has been suggested as a common pathology of polyQ diseases. Beyond clarification of a new foci of common polyQ pathologies by TERA/VCP/p97, this study even suggest a novel common pathology that could be shared by a wider range of neurodegenerative disorders, including polyQ diseases and TERA/VCP/p97-linked FTLD. Ubiquitin and TDP43-positive inclusion bodies are observed in the nuclei of cortical neurons in FTLD with TERA/VCP/p97 mutations [48] . The nuclear or cytoplasmic aggregates might disturb dynamics of TERA/VCP/p97 in the nuclei of neurons necessary for DSB repair, although the hypothesis should be further tested in the future. Again our results cast a light on the role of inclusion body because TERA/VCP/p97 was deprived by aggregation. The pathological significance of inclusion bodies or aggregation has been a focus of debate for over a decade. The previous concept that the inclusion body by itself possesses toxicity has been challenged after the observation that inclusion body-positive neurons are more resistant to mutant Htt [49] . We also observed that cell death is inversely related to inclusion bodies in primary neurons expressing mutant Htt [50] . However, the pathological role of the inclusion body remains ambiguous, because misfolded protein toxicity stemming from abnormal physiological protein interactions are inseparable from the aggregating structures of a disease protein. In our study, mutant polyQ proteins generally reduce the amount of TERA/VCP/p97 in the functional domains in cells, polyQ protein-mediated sequestration may also contributes to VCP pathology, at least as part of the disease process. These data seemed to support the later view. This idea was supported by the observation that the TERA/VCP/p97 dynamics in the nucleus was profoundly disturbed in inclusion body-positive cells ( Fig. 4 ). However, soluble protein or pre-aggregates of mutant polyQ proteins could also be toxic to the functions of TERA/VCP/p97. Actually, our live imaging showed a delay of TERA/VCP/p97 accumulation to DSB lesions even in cells without inclusion body ( Fig. 4 ). Moreover, the phenotype recovery of SCA1 and HD model flies was independent of aggregation ( Fig. 8 ). The discussion has not reach to a definite conclusion in this study as in many other cases of polyQ disease models, and probably both mechanisms will contribute to the pathology. Finally, although this study identified DNA damage repair, one of the multiple functions of TERA/VCP/p97, as a new common pathomechanism of polyQ diseases, it remains unclear to which extent DNA damage repair and other functions of TERA/VCP/p97 contribute to the polyQ disease pathology. Although our results suggested that contribution of TERA/VCP/p97-mediated ERAD was not large in neuronal pathology, it is not clear how our findings are correlated to autophagy. There are a number of evidences that activation of brain autophagy by chemicals attenuates toxicity of mutant Htt protein [51] , [52] , [53] and that a certain defect of autophagy contributes to other neurodegenerative disorders like Alzheimer’s disease [54] and Parkinson’s disease [55] . Meanwhile, a report showed that an mTOR inhibitor was effective for the muscle pathology but not brain pathology of HD [56] , and another group recently reported that a new mouse model of SCA6 did not show any change of autophagy in the brain [57] . In some preliminary studies, we also investigated macroautophagy in Purkinje cells of mutant Atxn1-KI mice by electron microscopy, but we have not been able to detect any changes. Moreover, multiple pathways like transcription, including PGC-1alpha, splicing, mitochondrial stress, ER stress and oxidative stress mediated by other common molecules may underlie degeneration. Therefore, we need fundamentally new technologies to quantitatively evaluate contribution of each pathomechanism (or pathway) to the pathology and symptom, and solution of such issues would greatly advance our understanding of the common pathomechanism of neurodegeneration and would help developing radical therapeutics based on the common pathology. Filter-binding assay HeLa cells were transfected by different amounts of Htt-103Q expression vector (0, 0.25, 0.5, 1, 2, 4 μg/4 × 10 −4 cells). After 36 h, cells were harvested and lysed with PBS-0.02% Nonidet P-40. The sup after centrifugation was filtrated by Durapore-PDVF (0.22 μm). The flow-through fraction was blotted with anti-VCP antibody (BD Transduction Laboratories, 1:1000). The signal intensities were corrected by GAPDH. ERAD analysis HEK 293 cells were plated in 24-well plates and transfected with pCl-neo-HA-CD3Δ (ERAD substrate) and polyQ disease protein expression vectors (HA-CD3Δ 0.06 μg; FLAG-VCP, 0.9 μg; Myc-polyQ, 0.6–0.9 μg; balanced by using a pCMV-3Tag-1A empty vector). After 24 h, the cells were subjected to treatment with or without CHX (final concentration, 100 μg ml −1 ). Thirty-six hours after the transfection, the cells were harvested directly into 50 μl of SDS sample buffer and processed for SDS–PAGE and immunoblotting for CD3Δ. The relative amount of HA-CD3Δ was measured using western blotting and was normalized by the amount of tubulin, which served as the internal controls. Film images were taken by a scanner and processed using the Image J software package ( http://rsb.info.nih.gov/ij/ ) to measure the band intensity. For ERAD assay with cortical neurons from Htt-111Q-KI mice [28] and ATXN1-154Q-KI mice [29] , primary neurons were prepared according to the method described previously [37] , [47] . The pCl-neo-HA-CD3Δ was transfected into neurons by lipofectamine LTX with Plus reagent (Invitrogen). ERAD analysis was performed using CHX as described above. ErbB2 analysis Cells transfected with GFP-ErbB2 and polyQ proteins and/or VCP (12-well dishes, glass coverslips; GFP-ErbB2, 0.3 μg; FLAG-VCP, 0.3 μg; Myc-polyQ, 0.4 μg) were incubated for 36 h and then fixed. The immunocytochemistry procedure mentioned above was performed to stain the Myc-polyQ and/or FLAG-VCP proteins. ATPase activity assay of VCP ATPase activity of VCP was assayed following the method reported previously [22] . Fresh brains dissected control and Htt-111Q-KI mice were homogenized in 20 mM HEPES (pH=7.5), 5 mM MgCl 2 , 2.5 mM DTT, 150 mM NaCl by Dounce homogenizer, sonicated (10 s × 3 times), and centrifuged at 20,000 g for 10 min. The sup was filtrated by 0.22 μm PVDF membrane (Milipore) and protein concentration was measured by BCA Protein Assay (Thermo). The extracts (5 mg ml −1 , 500 μl) were applied to high performance liquid chromatography (HPLC, Shimadzu) and fractionated by gel filtration chromatography (Superdex 200 10/300 GL, GE Healthcare) and ion exchange chromatography (DEAE-2SW, Tosoh). Each fraction (40 μl) was added to 50 μl reaction buffer (0.2 mM ATP (SIGMA), 20 mM HEPES (pH=7.5), 10 mM MgCl 2 ) and incubated for 120 min at 37 °C. After additional incubation for 30 min at 37 °C with BIOMOL GREEN (ENZO), phosphate ion released from ATP was assayed by measuring OD at 630 nm with plate reader (MULTISKAN ASCENT, Thermo). The values of phosphate ion were corrected with the amounts VCP in control and Htt-111Q-KI mice evaluated by western blot on a single membrane. Laser microirradiation Laser microirradiation and signal acquisition from damaged area were performed according to the method as described previously [58] . In the case of cell line, U2OS cells grown on 25-mm coverslips were treated with 2 μM Hoechst33258 (DOJINDO, Japan) for 20 min to sensitize the cells to DSBs. Using the software (AIM4.2, Carl Zeiss, Germany) of microscopy (LSM510META, Carl Zeiss, Germany), rectangle-shaped areas locating at cell nuclei were irradiated by UV laser (Maximum power: 30 mW, laser output: 75%, wavelength: 405 nm, iteration: 5, pixel time: 12 μs: zoom 6), and time-lapse images were obtained every 30 s. In the case of neuron, primary mouse cortical neurons cultured on Lab-Tek II Chambered Coverglass System (Thermo Fischer Scientific Inc, MA, USA) with the medium described above were similarly irradiated expect using zoom at 2, and signal acquisition was performed by immunocytochemistry with anti-VCP (Santa Cruz, H-120, 1:100) and anti-γH2AX (Millipore, JBW301, 1:1,000) antibodies at 1 h after irradiation. In both cases, region of interest matching exactly to the bleached area was determined using Adobe Photoshop CS3, and mean signal intensities per pixel of VCP protein were obtained from region of interest. Signal intensity was normalized by that of non-irradiated area, which was indicated as a normalized fluorescence unit. Lentiviral vectors were constructed by subcloning human full-length ataxin-1 cDNA or human huntingtin-exon1 cDNA from previously described plasmids [37] into Eco RI- Xba I and Xba I- Bam HI sites of pLVSIN-CMV Pur Vector (TaKaRa, Japan), respectively. DSB repair complex formation For interaction between VCP and L3MBTL1, HeLa cells (2 × 10 6 ) plated on 10 cm dishes were transfected with pCMV-FLAG-VCP described above, and incubated for 36 h. Cells were incubated for 1 h with 400 μg ml −1 of the radiomimetic drug Zeocin (Invitrogen) to induce DNA double strand breaks. After washing with PBS, cells were homogenized with 1 ml of TNE buffer and rotated at 4 °C for 2 h. Then, the solutions were centrifuged at 15,000 g for 15 min. The supernatant were incubated with 20 μl of protein G-sepharose beads (GE healthcare) for 2 h at 4 °C with rotation. After beads were removed, the lysates were incubated with 2.5 μg of anti-L3MBTL1 antibody overnight at 4 °C with rotation, followed by the incubation with protein G-sepharose for 2 h. The beads were washed five times with 500 μl of TNE buffer and resolved using SDS–PAGE sample buffer. Characterization of cytoplasmic vacuoles HeLa cells (1 × 10 5 ) were plated on glass coverslips in 12-well plates and transfected with a Myc-polyQ protein expression vector as described. Thirty-six hours after transfection, cells were fixed and stained with anti-Myc (Santa Cruz Biotechnology; 9E10) antibody, and the co-localization of Myc-polyQ with EGFP-LC3 (autophagosome marker) or DsRed containing an ER translocation sequence (KDEL) was examined. Cells possessing cytoplasmic vacuoles (classified by 10-μm diameter) were counted in 50 visual fields. Immunohistochemistry of polyQ disease model mice Fresh brains of heterozygous Htt-111Q-KI (48 weeks) [28] , ATXN1-154Q-KI (32 weeks) [29] , Htt-Tg (R6/2) mice [30] (12 weeks), ATXN7-92Q-Tg mice (33 weeks) [31] or AR-97Q-Tg mice [32] (13 weeks) were fixed in phosphate-buffered 4% paraformaldehyde and embedded in paraffin. Sections (thickness, 5–10 μm) were dewaxed in xylene and rehydrated using a descending ethanol series. Sections were boiled in 10 mM citrate buffer (pH 6.0) in a microwave oven three times and kept at room temperature for 30 min after the final boiling. Incubation in PBS containing 1% bovine serum albumin and 0.01% (v/v) Triton X-100 was performed for 30 min to block nonspecific binding. Samples were incubated overnight at 4 °C with a primary antibody, followed by incubation with a secondary antibody for 1 h at room temperature. After a 2-min DAPI treatment, the brains were mounted using Fluoromount and covered using coverslips. Cells were visualized using confocal microscopy (Zeiss LSM510). Primary antibodies and dilution conditions were as follows: anti-Htt antibody (HD1, 1:100), anti-ATXN1 antibody (11NQ, mouse 1:100), and anti-VCP antibody (Cell Signalling Technologies; rabbit, 1:100). Secondary antibodies and dilution conditions were as follows: Alexa Fluor 488-conjugated anti-mouse antibody (Molecular Probes; 1:1000) and Cy3-conjugated anti-rabbit antibody (Jackson; 1:1,000). Immunohistochemistry of human brain tissues Brains of genotype-diagnosed patients with HD or SCA1 were fixed in phosphate-buffered 4% paraformaldehyde and embedded in paraffin. Sections (thickness, 10 μm) were dewaxed in xylene and rehydrated using a descending ethanol series. Treatment and observation of the sections were similar to the methods for mouse brain tissues except for the antibody conditions. Primary antibodies and dilution conditions were as follows: anti-Htt antibody (HD1, 1:200), anti-ATXN1 antibody (H21, goat 1:100), and anti-VCP antibody (Becton Dickinson and Company; 1:200). Secondary antibodies and dilution conditions were as follows: Alexa Fluor 488-conjugated anti-mouse antibody (Molecular Probes; 1:1,000) and Cy3-conjugated anti-rabbit antibody (Jackson; 1:1,000). Ethics statement This study was performed in strict accordance with the recommendations in the Guide for the Care and Use of Laboratory Animals of the National Institutes of Health, and had been approved by the Committees on Human Ethics and Animal Experiments of the Tokyo Medical and Dental University (Number: 2011-22-3 and 0130225). How to cite this article: Fujita, K. et al . A functional deficiency of TERA/VCP/p97 contributes to impaired DNA repair in multiple polyglutamine diseases. Nat. Commun. 4:1816 doi: 10.1038/ncomms2828 (2013).